Tunably strained metallacycles enable modular differentiation of aza-arene C–H bonds 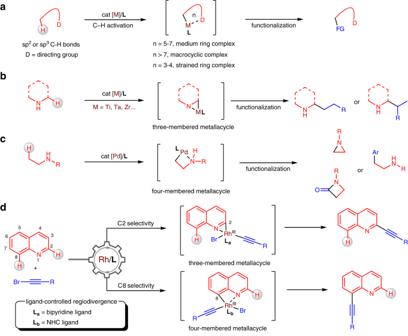Fig. 1: Background and discovery. aGeneral procedures for selective C–H activation assisted by directing groups.bα-Selective C–H functionalization of aliphatic amines via metallaaziridine intermediates.cβ-Selective C–H functionalization of aliphatic amines via four-membered metallacycles.dModular differentiation of quinolines by tunable three- and four-membered ring cyclometallation. The precise activation of C–H bonds will eventually provide chemists with transformative methods to access complex molecular architectures. Current approaches to selective C–H activation relying on directing groups are effective for the generation of five-membered, six-membered and even larger ring metallacycles but show narrow applicability to generate three- and four-membered rings bearing high ring strain. Furthermore, the identification of distinct small intermediates remains unsolved. Here, we developed a strategy to control the size of strained metallacycles in the rhodium-catalysed C−H activation of aza-arenes and applied this discovery to tunably incorporate the alkynes into their azine and benzene skeletons. By merging the rhodium catalyst with a bipyridine-type ligand, a three-membered metallacycle was obtained in the catalytic cycle, while utilizing an NHC ligand favours the generation of the four-membered metallacycle. The generality of this method was demonstrated with a range of aza-arenes, such as quinoline, benzo[ f ]quinolone, phenanthridine, 4,7-phenanthroline, 1,7-phenanthroline and acridine. Mechanistic studies revealed the origin of the ligand-controlled regiodivergence in the strained metallacycles. Due to the near universal advantage of C − H bonds in organic molecules, the C − H activation strategy provides an opportunity to functionalize any carbon centre in an atom-economical and streamlined way [1] , [2] , [3] , [4] , [5] , [6] , [7] , [8] , [9] , [10] . Because organic molecules typically contain multiple C − H bonds with comparable strengths and steric environments, regiocontrol has been a long-standing challenge within this type of chemistry [11] . The differentiation of C − H bonds is traditionally dominated by steric and electronic effects [12] , and there have been considerable efforts to utilize directing groups in less constrained molecules (Fig. 1a ) [13] , [14] , [15] , [16] , [17] . Directed C − H activation is thermodynamically favoured through conformationally rigid five-, six-, and seven-membered metallacyclic intermediates. Several elegant methods have been exploited to achieve the meta - and para -selective C − H activation of arenes through chelation-assisted macrocyclic complexes by directing groups [18] , [19] , [20] , [21] , [22] . Despite these advances, the generation of highly strained metallacycles in directed C − H activation remains much desired but more challenging. Fig. 1: Background and discovery. a General procedures for selective C–H activation assisted by directing groups. b α-Selective C–H functionalization of aliphatic amines via metallaaziridine intermediates. c β-Selective C–H functionalization of aliphatic amines via four-membered metallacycles. 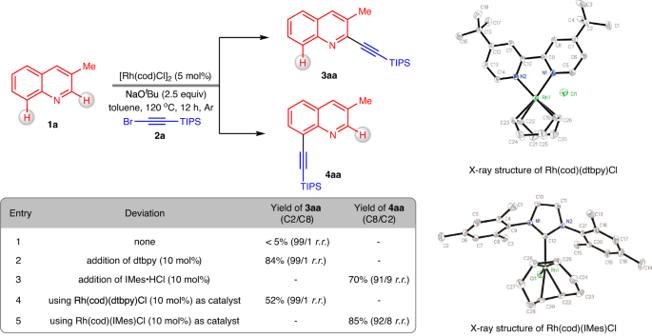Fig. 2: Effect of the ligands on reactivity and regioselectivity. The regioselectivity ratio (r.r.) was determined by GC‒MS analysis of the reaction mixtures. dtbpy = 4,4’-di-tert-butyl-2,2’-bipyridine. IMes =1,3-bis (2,4,6-trimethylphenyl)−1,3-dihydro-2H-imidazol-2-ylidene. d Modular differentiation of quinolines by tunable three- and four-membered ring cyclometallation. Full size image Substantial progress has been made regarding the C–H activation of aliphatic amines through strained metallacycles, allowing for site-selective functionalization at the α or β position of the amino group in one catalytic step [23] , [24] . Early transition metals, including titanium, tantalum and zirconium, enable the hydroaminomethylation of alkenes with unprotected N-heterocycles and amines through metallaaziridine intermediates, affording either linear or branched products (Fig. 1b ) [25] , [26] , [27] , [28] , [29] , [30] . A series of C–H functionalizations of aliphatic amines have been developed by palladium catalysis, showing β-selectivity through a four-membered ring cyclopalladation pathway (Fig. 1c ) [31] , [32] , [33] . Compared to small aliphatic metallacycles, the formation of benzo-fused analogues comes with larger ring strain. We questioned whether such metallacycles could be generated through chelation with inherent nitrogen atoms in aza-arenes. Furthermore, switching the ring size in a unifying system to differentiate of two C–H bonds would likely have a broad impact on the continued advancement of this field. As a representative example of bicyclic aza-arenes, quinoline contains seven C − H bonds in the pyridine (C2 to C4) and benzene (C5 to C8) cores that can be functionalized [34] , [35] . Structural modification of the pyridine ring has been achieved by taking advantage of strong electronic and steric bias [36] , [37] , [38] , [39] , [40] , [41] , [42] , [43] . 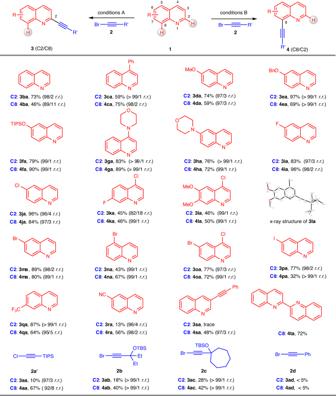Fig. 3: Substrate scope of the regiodivergent C–H alkynylation of quinolines at the C2 and C8 positions. Reaction Conditions A: [Rh(cod)Cl]2(5 mol%), dtbpy (10 mol%),1(0.20 mmol, 1.0 equiv),2(0.50 mmol, 2.5 equiv), NaOtBu (0.50 mmol, 2.5 equiv), 1 mL of toluene, 120 °C, 12 h, under argon. Reaction Conditions B: [Rh(cod)(IMes)Cl (10 mol%),1(0.20 mmol, 1.0 equiv),2(0.50 mmol, 2.5 equiv), NaOtBu (0.50 mmol, 2.5 equiv), 1 mL of toluene, 120 °C, 12 h, under argon. r.r. values were determined by GC‒MS analysis of the reaction mixture. An indirect route to access the benzene core involves the oxidation of quinoline to its N -oxide, followed by oxygen-directed C − H functionalization and subsequent reduction to the desired products [44] , [45] , [46] . To provide more flexibility to access the benzene core, metal clusters and dimers such as Os 3 (CO) 10 [47] , Ru 3 (CO) 12 [48] , and Rh 2 (OAc) 4 [49] have been employed in C − H activation through bridged metal-metal bonds. Enabled by bimetallic palladium catalysis, Yu and coworkers also designed a class of remote-directing template for differentiation of C − H bonds (C5-C7) at the benzene core of quinolines [50] , [51] , [52] , [53] . Here, we report the successful realization of a strategy for regiodivergent C–H activation of aza-arenes enabled by tunably strained metallacycles under monomeric rhodium catalysts (Fig. 1d ). The precise differentiation of two C–H bonds proceeds through a switchable three- or four-membered-ring cyclometallation pathway by just tuning the structure of the ligands. Incorporation of alkyne motifs into aza-arenes are valuable transformations to build C–C bonds and provide a versatile handle for further modifications. Reaction design As shown in Fig. 2 , we first evaluated the reaction of 3-methylquinoline ( 1a ) with (bromoethynyl)triisopropylsilane ( 2a ). After treatment of [Rh(cod)Cl] 2 (5 mol%) with NaO t Bu (2.5 equiv) at 120 °C under an Ar atmosphere in toluene, the desired product 3aa was generated in trace amounts after 12 h (entry 1). After screening a variety of ligands for optimization (for the details of the reaction optimization, see the Supplementary Information ), the optimized conditions for C2-alkynylation were determined, using 10 mol% dtbpy as a ligand. Under these conditions, product 3aa was afforded in 84% yield, showing 99/1 r.r . of the C2 to C8 positions (entry 2). Interestingly, employing NHC ligands [54] resulted in a preference for C8 selectivity, and the use of IMes·HCl led to the formation of product 4aa in 70% yield (C8/C2 = 91/9 r.r .) (entry 3). Employment of [Rh(cod)Cl] 2 with the optimal ligands resulted in the production of two rhodium complexes, Rh(cod)(dtbpy)Cl and Rh(cod)(IMes)Cl, both of which were unambiguously assigned by X-ray crystallography. Utilizing the pregenerated Rh(cod)(dtbpy)Cl as the catalyst showed a much lower reactivity than the in situ generation of the catalyst (entry 4). In contrast, the use of Rh(cod)(IMes)Cl as the catalyst improved the generation of 4aa to 85% yield with 92/8 r.r . (entry 5). Fig. 2: Effect of the ligands on reactivity and regioselectivity. The regioselectivity ratio (r.r.) was determined by GC‒MS analysis of the reaction mixtures. dtbpy = 4,4’-di-tert-butyl-2,2’-bipyridine. IMes =1,3-bis (2,4,6-trimethylphenyl)−1,3-dihydro-2H-imidazol-2-ylidene. Full size image Scope of the methodology The scope of the regiodivergent C–H alkynylation was then examined (Fig. 3 ). In general, a series of commercially available quinolines with varied substituents reacted smoothly with bromoalkyne 2a , yielding two types of alkynylation products under reaction conditions A and B. The reaction of quinoline ( 1b ) with bromoalkyne 2a underwent C2- and C8-selective C–H alkynylation, providing products 3ba (98/2 r.r .) and 4ba (89/11 r.r .) with excellent regioselectivities. The quinolines that incorporated electron-donating groups, including phenyl ( 1c ), ether ( 1d-e ), silyloxy ( 1 f ), and amino ( 1g-h ) groups, at different positions were readily tolerated with bromoalkyne 2a to produce the corresponding products 3ca - ha and 4ca - ha with excellent regioselectivity under both reaction conditions. Halide-containing quinolines 1i-p bearing F, Cl, Br, and even I motifs were compatible with the generation of both the C2 and C8 alkynylation products. Among them, substrates 1k - l containing substituents at the C7 position did not sterically block the reaction at the C8 position. Quinoline 1q bearing a CF 3 group was also compatible with both sets of reaction conditions, affording 3qa and 4qa in 87% and 64% yields, respectively. The use of 6-cyanoquinoline ( 1r ) under condition A became too sluggish to provide product 3ra , but this substrate did not interfere with productive C–H alkynylation at the C8 position. Quinoline 1 s , containing a phenylethynyl motif at the C3 position inhibited the reactivity at the C2 position but enabled C8-selective C–H alkynylation to generate product 4sa . As a bidentate nitrogen ligand, 2,2′-biquinoline ( 1t ) could also engage under reaction conditions B to deliver the expected products 4ta in a good yield. We further explored the scope of alkynyl bromides with quinoline 1a . Compared to reagent 2a , the reaction of TIPS-protected ethynyl chloride ( 2a’ ) showed much lower reactivity in both reaction systems. Alkynylation with propargyl silyl ethers 2b-c afforded the desired products in significantly lower yields, but maintained the excellent regioselectivity. Alkynyl bromides 2d with a less sterically hindered phenyl group were problematic under both reaction conditions, and the corresponding products 3ad and 4ad were observed in only trace amounts. The poor outcomes are attributed to the lower stability of these bromoalkynes without TIPs group under the reaction conditions [55] , [56] , [57] , [58] , [59] . Fig. 3: Substrate scope of the regiodivergent C–H alkynylation of quinolines at the C2 and C8 positions. Reaction Conditions A: [Rh(cod)Cl] 2 (5 mol%), dtbpy (10 mol%), 1 (0.20 mmol, 1.0 equiv), 2 (0.50 mmol, 2.5 equiv), NaO t Bu (0.50 mmol, 2.5 equiv), 1 mL of toluene, 120 °C, 12 h, under argon. Reaction Conditions B: [Rh(cod)(IMes)Cl (10 mol%), 1 (0.20 mmol, 1.0 equiv), 2 (0.50 mmol, 2.5 equiv), NaO t Bu (0.50 mmol, 2.5 equiv), 1 mL of toluene, 120 °C, 12 h, under argon. r.r. values were determined by GC‒MS analysis of the reaction mixture. Full size image Other aza-arenes commonly featured in bioactive molecules and functional materials were next targeted. Benzo[ f ]quinoline ( 5a ) was first employed in the catalytic systems and gave desired products 6aa and 7aa at the C3 and C5 positions, respectively (Fig. 4a ). Phenanthridine ( 5b ), the key aromatic unit of many DNA stains, underwent regiodivergent C–H alkynylation at the C6 and C4 positions in high yields with excellent selectivities (Fig. 4b ). Treatment of 4,7-phenanthroline ( 5c ) containing two azine motifs under reaction conditions A afforded a promising mixture of mono- and di-substituted products 6ca and Fig. 4: Regiodivergent C–H alkynylation of diverse aza-arenes. a C–H alkynylation of benzo[ f ]quinolone ( 5a ). b C–H alkynylation of phenanthridine ( 5b ). c C–H Alkynylation of 4,7-phenanthroline ( 5c ). d C–H alkynylation of 1,7-phenanthroline ( 5d ). e C–H alkynylation of acridine ( 5e ). Full size image 6ca’ with a high regioselectivity (Fig. 4c ). Similarly, the two products 7ca and 7ca’ were also generated under reaction conditions B with excellent regioselectivity. Notably, the products with one or two alkynyl motifs could be separated by column chromatography on silica. When 1,7-phenanthroline ( 5d ) was treated under reaction conditions A, C–H alkynylation occurred at the C8 position. However, an unusual C10-functionalized product 7da’ was obtained under reaction conditions B, indicating that C–H metalation process preferred to undergo five-membered metallacyclic intermediate (Fig. 4d ). Finally, acridine ( 5e ), bearing two C–H bonds (C4 and C5) for activation, gave only the monosubstituted product 7ea in 85% yield with complete selectivity (Fig. 4e ). Synthetic applications To showcase the synthetic utility of this discovery, gram-scale reactions of quinolone 1j were first performed under both reaction conditions, and products 3ja and 4ja were isolated in 96% and 85% yields without erosion of the regioselectivity (Fig. 5a ). Further derivatizations of 3ja were achieved with synthetically useful intermediate 8 , which was obtained in 70% yield by the TBAF-mediated removal of the TIPS group. For instance, hydrogenation of 8 under 1 atm of hydrogen with a catalytic amount of Pd/BaCO 3 yielded alkylation product 9a in high yield. The use of the Wilkinson catalyst for hydrogenation allowed for the chemoselective synthesis of olefin 9b . The terminal triple bond in 8 could be effectively transformed into an internal bond to provide product 9c in nearly quantitative conversion through the Sonogashira reaction. Ag catalysis of the reaction of 8 with NBS formed bromination product 9d in excellent yield. In addition, alkyne 8 was easily converted to triazole 9e with BnN 3 via a copper-catalysed click reaction. Based on diverse alkyne conversion, our strategy provides a simple and distinct way to construct a number of pharmaceutically relevant compounds and materials. The reaction of quinoline 10 under Conditions B furnished C2-alkynylation, and further removal of the TIPS group provided Compound 11 in good yield, acting as a core framework for the tautomerase inhibitor (Fig. 5b ). As a key intermediate for the synthesis of montelukast, Compound 13 was rapidly prepared from quinoline 12 by C2-selective C–H alkynylation with bromoalkyne 2a , further removal of the TIPS group and reduction with the Wilkinson catalyst under 1 atm of hydrogen (Fig. 5c ). Compound 15 is a key intermediate in the synthesis of BN-dibenzo[a,o]picene, and 3,8-dibromo-4,7-phenanthroline ( 14 ) must be pregenerated through multistep synthesis from 5c to access this molecule by Sonogashira coupling (Fig. 5d ) [60] . Notably, this molecule can be prepared in an atom- and step-economic way, further indicating the value of the developed method. Fig. 5: Synthetic applications of regiodivergent C–H alkynylation. a Gram-scale preparation of 3ja and 4ja and their derivatizations. b Application of the process to the synthesis of potent tautomerase inhibitors. c Application of the process to the synthesis of montelukast. d Application of the process to the synthesis of BN-dibenzo[a,o]picene. Full size image Mechanistic study In order to gain insights into the reaction pathways and origin of positional selectivity, density functional theory (DFT) calculations were performed using the reaction of quinoline 1b and alkynyl bromide 2a as the model (Fig. 6 ). The reaction initially commences by the formation of 1b and the ligand bound Rh(I) intermediate INT1A , which is set as the relative zero point of the Gibbs free energy. The previous reported Rh(I)-involved C–H activation by oxidative addition might be a reversible process with an activation energy barrier of 26.2 kcal mol −1 (for the details of the computational data, see the Supplementary Information ) [36] , [37] , [38] . Comparably, INT1A more favorably coordinates with 2a to generate INT2A , which then undergoes C–Br bond oxidative addition to afford Rh(III) species INT3A . In the case of the dtbpy ligand, the C–Br oxidative addition through transition state TS3A-dtbpy was calculated to have an activation free energy of 27.6 kcal mol −1 . This step is the rate-determining step in the catalytic cycle. The resulting intermediate INT3A-dtbpy occurs C2–H metalation through a t butoxide-assisted deprotonation with a 25.8 kcal mol −1 energy barrier [61] , [62] , [63] , [64] , [65] , [66] . Further reductive elimination and ligand exchange yield the desired products with high selectivity and regenerates INT1A to complete the catalytic cycle. For the IMes ligand, the C–Br bond oxidative addition to the Rh(I) center from INT2A-IMes has an activation energy of 26.7 kcal mol −1 , which shows a comparable energy barrier with the subsequent C–H activation (26.1 kcal mol −1 ). In the following C − H metalation, IMes ligand favors C8 selective transition state TS4B-IMes . Fig. 6: Calculated energy profiles of the regiodivergent C–H alkynylation of 1b with 2a. 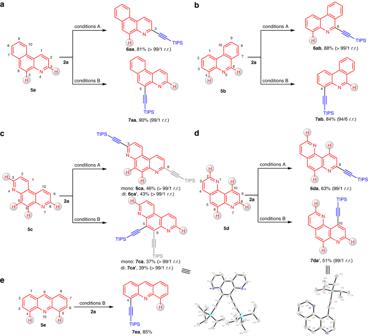Fig. 4: Regiodivergent C–H alkynylation of diverse aza-arenes. aC–H alkynylation of benzo[f]quinolone (5a).bC–H alkynylation of phenanthridine (5b).cC–H Alkynylation of 4,7-phenanthroline (5c).dC–H alkynylation of 1,7-phenanthroline (5d).eC–H alkynylation of acridine (5e). a The proposed catalytic cycles with different ligands. b The key transition states in the catalytic cycle. Full size image As shown in Fig. 7 , extensive computational studies on different site selectivity were also carried out. The molecular electrostatic potential map was used to analysis the possible nucleophilic sites of quinoline 1b (Fig. 7a ). Quantitatively, the natural population analysis of 1a shows that C2 has an atomic charge of −0.069e, which is less charged than C8 (−0.192e), illustrating C2 − H is relative electron deficient and more prone to C − H metallization with electron-rich rhodium catalyst (Supplementary Data 1 ). Inspecting computed electrostatic potential maps of Rh − dtbpy and Rh − IMes , the dtbpy ligand exhibits more electron-donating ability than IMes, allowing INT3A-dtbpy to preferentially react with the C2 position of 1b . The energy barrier of the rhodacycle transition state TS4A-dtbpy that delivers the three-membered intermediate INT4A-dtbpy is 8.2 kcal mol −1 lower than that of the competing transition state TS4B-dtbpy that leads to the INT4B-dtbpy (Fig. 7b ). This energy difference is consistent with the experimentally excellent site selectivity of 3ba . Without the nitrogen chelation, transition states TS4C-dtbpy and TS4D-dtbpy have activation barriers of 42.0 and 43.9 kcal mol −1 , respectively. Such high computed energies are mainly ascribed to the intrinsic inertness of the C − H bonds at the C2 and C8 position of quinoline, indirectly illustrating the importance of the directing group. The directed C–H metalation transition state through TS4B-IMes has an activation Gibbs free energy of 26.1 kcal mol −1 , which is 17.3 kcal mol −1 lower than the same process through TS4A-IMes (26.1 and 43.4 kcal mol −1 ) and 11.2 kcal mol −1 lower than the original nucleophilic attack at quinoline C2 position through TS4C-IMes (26.1 and 37.3 kcal mol −1 ). In addition, the steric maps around the Rh(III) centre with IMes ligand were analyzed based on the SambVca 2.1 tool (Fig. 7c ) [65] , [66] . All transition states adopt trigonal bipyramidal geometries, where Br atom and O t Bu group occupy the two vertex positions and the IMes ligand in the NW quadrant of the steric map extends to the NE and SW quadrants. In disfavored transition state TS4A-IMes , bicyclo 3-4 fused rhodacycle enables the Rh−C bond formation to occur in the SW quadrant, which suffers from significant repulsion with Mes group of the carbene ligand. The favored transition state TS4B-IMes is a bicyclo 4-4 fused rhodacycle, the expansion of ring size makes the quinoline backbone more horizontally extended and reduce the steric hindrance between quinoline and TIPS group, thereby effectively lowering the energy barrier of TS4B-IMes . In TS4C-IMes and TS4D-IMes , Rh−N bond distances are elongated to 2.85 and 3.57 Å, respectively, indicating nitrogen atom in 1b is not anchored around the Rh(III) centre. Taken together, the electronic and steric effects account for the tunability of the strained metallacycles, achieving different positional selectivity [67] , [68] . Fig. 7: The origin of the site selectivity. a Molecular electrostatic potential map of 1b, Rh−dtbpy , and Rh−IMes . b Key transition states for the different site selectivities. c Steric maps of the Rh(III) transition states TS4A-IMes, TS4B-IMes, TS4C-IMes , and TS4D-IMes . Full size image In conclusion, the present results demonstrate an important initial advance in C–H activation through a benzo-fused three- or four-membered ring cyclometallation pathway in a switchable mode. This chemistry provides a unique tool for the functionalization of high-value aza-arenes with divergent site selectivities controlled by ligands. The switch of the positional selectivity through strained metallacycles fills a major methodological gap in directed C–H activation. We anticipate that other transformations based on this strategy could be exploited for molecular editing of aza-arene C–H bonds, providing inspiration for the design of new tactics to produce complex bioactive molecules, natural products and functional materials. 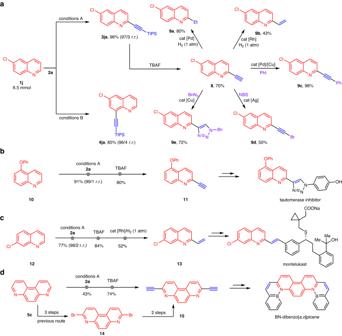Fig. 5: Synthetic applications of regiodivergent C–H alkynylation. aGram-scale preparation of3jaand4jaand their derivatizations.bApplication of the process to the synthesis of potent tautomerase inhibitors.cApplication of the process to the synthesis of montelukast.dApplication of the process to the synthesis of BN-dibenzo[a,o]picene. 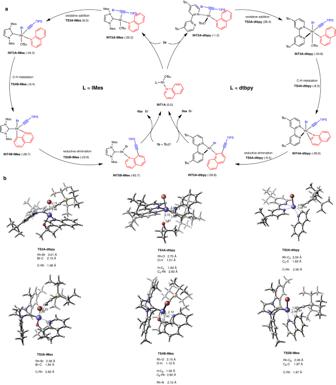Fig. 6: Calculated energy profiles of the regiodivergent C–H alkynylation of 1b with 2a. aThe proposed catalytic cycles with different ligands.bThe key transition states in the catalytic cycle. 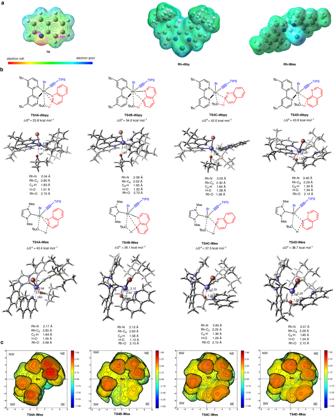Fig. 7: The origin of the site selectivity. aMolecular electrostatic potential map of1b,Rh−dtbpy, andRh−IMes.bKey transition states for the different site selectivities.cSteric maps of the Rh(III) transition statesTS4A-IMes,TS4B-IMes,TS4C-IMes, andTS4D-IMes. Due to slight variations in experimental protocols for all the processes we present, we refer the reader to the Supplementary Methods for experimental details.